Hydride ions in oxide hosts hidden by hydroxide ions The true oxidation state of formally ‘H − ’ ions incorporated in an oxide host is frequently discussed in connection with chemical shifts of 1 H nuclear magnetic resonance spectroscopy, as they can exhibit values typically attributed to H + . Here we systematically investigate the link between geometrical structure and chemical shift of H − ions in an oxide host, mayenite, with a combination of experimental and ab initio approaches, in an attempt to resolve this issue. We demonstrate that the electron density near the hydrogen nucleus in an OH − ion (formally H + state) exceeds that in an H − ion. This behaviour is the opposite to that expected from formal valences. We deduce a relationship between the chemical shift of H − and the distance from the H − ion to the coordinating electropositive cation. This relationship is pivotal for resolving H − species that are masked by various states of H + ions. Hydrogen is a ubiquitous element that exhibits various types of bonding in materials [1] , [2] , [3] . For example, hydrogen reacts with electropositive metal elements to form metal hydrides, in which hydrogen is treated formally as H − ions, whereas in most metal oxides, hydrogen forms OH − ions and is formally in the H + state. Both H − and H + can be doped into polar semiconductor hosts and the stability of each species is controlled by Fermi level [3] . Recently, incorporating H − ions into metal oxides and mixed-anion compounds has attracted much attention as a new approach to modify the physical and chemical properties of inorganic materials [4] , [5] , [6] , [7] , [8] , [9] , [10] , [11] , [12] including high-temperature superconductors [9] , [10] . Such materials are accessible by new chemical processes using metal hydride as a strong reducing reagent and/or hydrogen source. The effects of H − incorporation include antiferromagnetic coupling of two neighbouring cations [5] , [6] , tuning of ionic size of halide ion sites by hydride ion-substitution [9] , [10] , stabilization of high-symmetry polymorphic phases [11] and hosts for fast ion diffusion [11] , [12] . Furthermore, the large negative redox potential of H 2 /H − (−2.2 V with respect to H + /H 2 (SHE) and 0.3–0.5 V with respect to Li + /Li (ref. 13 )) may not only be useful for employing H − as a reductant in organic and electrochemical reactions [14] but may also facilitate redox reactions inside materials containing H − ions. An example of the latter has been reported for H − ion-doped mayenite [15] , [16] , [17] , [18] , [19] , [20] , [21] , [22] , [23] , [24] , [25] , [26] , in which H − ions are photochemically converted to protons by releasing carrier electrons [15] , [16] , [17] . A similar photochemical conversion process is also found on the surface of MgO (ref. 27 ). Nevertheless, whether ‘H − ’ ions can be routinely incorporated in oxide hosts and, if so, whether they indeed possess the chemical state of H − ions, is still debated. These questions frequently arise in connection to the chemical shifts of 1 H nuclear magnetic resonance (NMR) spectroscopy in non-metals, which exhibit values that are typical for H + , for example, ~+5 p.p.m. with respect to tetramethylsilane (TMS) [11] , [17] , [18] , whereas ‘metallic’ hydrides, such as TiH 2 , exhibit large negative shifts [28] . To resolve this controversy regarding the chemical shifts of H − ions in 1 H NMR spectra, here we systematically investigate the effect of the local environment of H − and OH − ions in an oxide host, mayenite, on chemical shift with a combination of experimental and ab initio approaches as well as re-examining published data. We deduce that the distance from the H − ion to the coordinating cation is a simple but essential parameter that determines the chemical shift of H − via a linear relationship. This relationship allows the overlapping NMR signatures of H − and H + ions to be separated from each other, which we demonstrate using H − ions diluted in calcium phosphate apatite as an example. Incorporation of H − and OH − ions into mayenites The structural formula of mayenite is [ M 24 Al 28 O 64 ] 4+ ·4 X − , where the brackets correspond to the lattice framework of a unit cell with a space group I 3 d , and M is Ca (refs 15 , 16 , 17 , 18 , 19 , 20 , 21 , 22 , 23 , 24 , 25 ) or Sr (ref. 26 ). A framework of AlO 4 tetrahedra, together with Ca 2+ or Sr 2+ ions embedded in it, forms cages that can accommodate various ‘extraframework’ anions indicated by 4 X − (see Fig. 1 ). Both Ca- and Sr-mayenites (described as C12A7 and S12A7, respectively) can theoretically accommodate up to four H − or OH − ions (4 X − hereafter) per 12 cages of the unit cell. Five mayenite samples incorporating different extraframework anionic species ( X − =OH − , H − and e − ) with concentrations close to theoretical maxima were prepared. The chemical compositions of these samples were determined using diffractometries, NMR spectroscopy and supporting analysis. 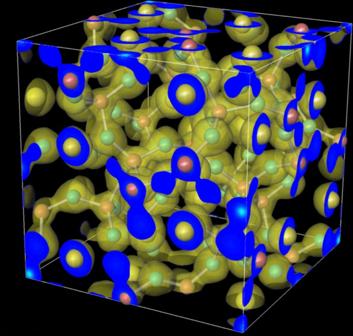Figure 1: Crystal structure of C12A7. The electron density isosurface (0.5 × 10−6e·pm−3) in [Ca24Al28O64]4+·4e−obtained by maximum entropy method analysis and superposed on the atomic structure of the unit cell determined by Rietveld analysis (Ca: yellow; Al: red; O: cyan). The framework charge can also be compensated by incorporation of anions into cages, whose occupancy is one-sixth in the case of divalent anions such as O2−and S2−, and one-third in the case of monovalent anions such as F−, OH−and H−. (see the Methods section) Figure 1: Crystal structure of C12A7. The electron density isosurface (0.5 × 10 −6 e ·pm −3 ) in [Ca 24 Al 28 O 64 ] 4+ ·4e − obtained by maximum entropy method analysis and superposed on the atomic structure of the unit cell determined by Rietveld analysis (Ca: yellow; Al: red; O: cyan). The framework charge can also be compensated by incorporation of anions into cages, whose occupancy is one-sixth in the case of divalent anions such as O 2− and S 2− , and one-third in the case of monovalent anions such as F − , OH − and H − . 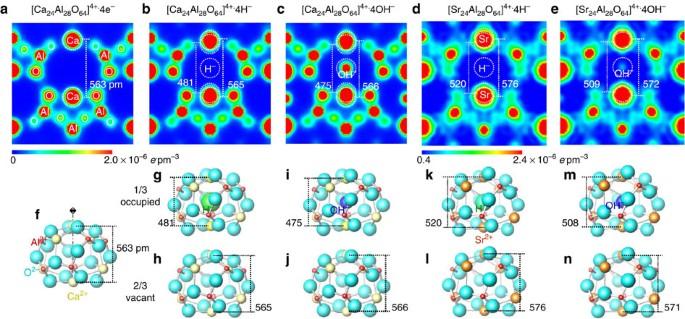Figure 2: Incorporation of H−and OH−anions into mayenites observed by X-ray diffraction. Upper row shows maximum entropy method electron density maps in the {400} planes for C12A7:e−(a), C12A7:H−(b), C12A7:OH−(c), S12A7:OH−(d) and S12A7:OH−(e) samples. Distances (pm) between the two pole Ca2+ions on theS4axes, as determined by Rietveld analysis, are indicated on the maps. The lower row shows the geometrical structures of the cages (Ca2+: yellow; Sr2+: orange; Al3+: red; O2−: cyan; H−: green; OH−: blue) and the corresponding Ca–Ca and Sr–Sr distances. Structures of the occupied and vacant cages are shown separately for C12A7:H−(g: occupied;h: vacant) and C12A7:OH−(i: occupied;j: vacant), S12A7:OH−(k: occupied;l: vacant) and S12A7:OH−(m: occupied;n: vacant) systems. Full size image Figure 2 displays the results obtained from Rietveld analysis and electron density analysis with the maximum entropy method (MEM) of synchrotron X-ray diffraction (XRD) data measured for the five samples. When comparing the three electron density maps for the C12A7 ( Fig. 2a–c ), only OH − ions are clearly observed in the cages, whereas the cage centres in samples containing extraframework e − and H − appear to be empty. However, the presence of H − is manifested by another feature in the density maps. In particular, the electron density for Ca 2+ ions is spherical in the C12A7:e − sample, whereas it has an ellipsoidal shape elongated along the S 4 axis in the samples containing H − and OH − ions. This elongation is interpreted as a superposition of the densities of Ca 2+ ions located at the poles of the vacant cages and those occupied by H − or OH − anions. In both cases, the concentration ratio of the vacant cages to the occupied ones is very close to the ideal ratio of 2:1 (refs 22 , 24 , 26; see Supplementary Tables 1–3 , and Supplementary Note 1 ), which allows us to calculate the displacement of two Ca 2+ ions at the cage poles inwards along the S 4 axis to be ~40 pm with respect to their sites in an empty cage in both C12A7:H − and C12A7:OH − . A similar effect is observed in S12A7 ( Fig. 2d,e ), where the extraframework H − and OH − ions induce the displacement of the pole Sr 2+ ions inwards by ~30 pm (see Supplementary Tables 4 and 5 , and Supplementary Note 2 ). Again the MEM analysis directly resolves OH − ions in the cage centre, but not H − ions. However, neutron powder diffraction (NPD) of the S12A7:H − sample implied almost theoretical maximum occupation of hydrogen in cages (see Supplementary Table 6 and Supplementary Note 3 ), confirming the presence of H − in the cages. Figure 2: Incorporation of H − and OH − anions into mayenites observed by X-ray diffraction. Upper row shows maximum entropy method electron density maps in the {400} planes for C12A7:e − ( a ), C12A7:H − ( b ), C12A7:OH − ( c ), S12A7:OH − ( d ) and S12A7:OH − ( e ) samples. 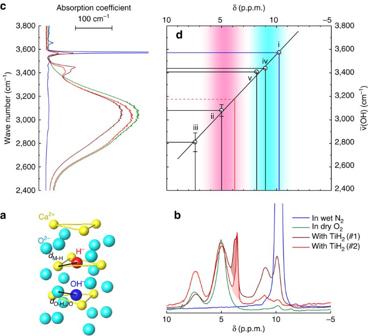Figure 6: H−ions in apatites. (a) Local structure around the channel in apatite, showing the coordinating ions with OH−and H−ions. (b)1H−magic-angle-spinning nuclear magnetic resonance (NMR) spectra collected in apatite samples annealed in wet N2(indicated by blue lines), in dry O2(orange) and with TiH2(brown and red). Filled areas highlight the signals assigned to H−ions. (c) Infrared transmission spectra measured for the same set of samples. (d) Correlation between chemical shifts (δiso) in the NMR spectra and wavenumbers in the infrared spectra. Blue and red shaded areas indicate chemical shift ranges predicted using thedM–HanddO–H…Ocorrelations withδiso(H−) andδiso(H+), respectively, given inFig. 4and equation 1. Distances (pm) between the two pole Ca 2+ ions on the S 4 axes, as determined by Rietveld analysis, are indicated on the maps. The lower row shows the geometrical structures of the cages (Ca 2+ : yellow; Sr 2+ : orange; Al 3+ : red; O 2− : cyan; H − : green; OH − : blue) and the corresponding Ca–Ca and Sr–Sr distances. Structures of the occupied and vacant cages are shown separately for C12A7:H − ( g : occupied; h : vacant) and C12A7:OH − ( i : occupied; j : vacant), S12A7:OH − ( k : occupied; l : vacant) and S12A7:OH − ( m : occupied; n : vacant) systems. Full size image The distances between the pole cations in C12A7:OH − and S12A7:OH − differ by 33 pm, which is consistent with the difference between ionic diameters defined by Shannon [29] : 242 and 212 pm for Sr 2+ (VII) and Ca 2+ (VII) (in this case, each cation is coordinated with six framework O 2− ions and one OH − ion), respectively. This agreement indicates that an OH − ion is sandwiched by the two pole cations in both C12A7 and S12A7 and its effective ionic radius is 132±2 pm, which, again, coincides with the value defined for OH − (II) [29] . Similarly, using the distance between the metal cation and hydride ion ( d Ca–H =240 pm and d Sr–H =266 pm), the ionic radius of an H − ion is 134±2 pm, which is slightly larger than the radius of F − (II) (128.5 pm) and almost the same as the radius of O 2− (II) (135 pm). This evaluation agrees with the generally accepted trend that the radius of an H − ion is nearly the same or slightly larger than that of an F − ion and increases with increasing electropositivity of the coordinating cation [29] . Another important geometrical parameter is the distance between the oxygen atom of the OH − ion and an O 2– ion ( d O–H…O ), which forms a hydrogen bond [1] , [30] , [31] . Taking into account the average displacements of OH − ions from the cage centre as estimated from the thermal parameters of Rietveld analysis, these distances are evaluated to be 313 and 322 pm in C12A7 and S12A7, respectively. These d O–H…O values are much larger than those in various other host materials, suggesting that these OH − ions have only weak hydrogen bonds. Nevertheless, these d O–H…O values are consistent with an empirical relation [1] linking d O–H…O and O–H stretching mode frequency (3,560 cm –1 for C12A7 (ref. 25 ) and 3,650 cm –1 for S12A7 (ref. 26 )). Important structural parameters of the samples are summarized in Table 1 . Table 1 Structural and electronic data. Full size table NMR chemical shifts The magic-angle-spinning (MAS) technique is indispensable for NMR characterization of a solid material. However, information about the anisotropy of the electron density around the nucleus and dipole–dipole interactions is sacrificed to improve spectrum resolution. 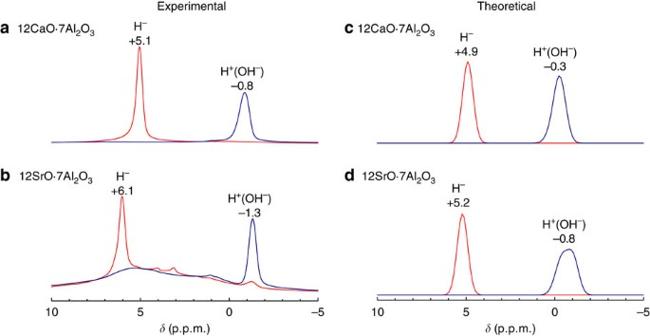Thus, the isotropic chemical shift, δ iso , is a principal parameter to characterize the chemical states of hydrogen [32] , [33] . Figure 3:1H nuclear magnetic resonance (NMR) spectroscopy. Experimental1H-magic-angle-spinning NMR spectra for (a) C12A7:H−(red line) and C12A7:OH−(blue line), and (b) S12A7:H−(red line) and S12A7:OH−(blue line) samples, and corresponding theoretical spectra for (c) C12A7 and (d) S12A7 systems. Broad signals between +7 and −2 p.p.m. in the experimental spectra of S12A7 are attributed to adsorbed water and hydroxide impurities. Figure 3 shows 1 H-MAS-NMR spectra measured for H − and H + (extraframework OH − ion) in C12A7 and S12A7. The H − ion has a peak at +5.1 p.p.m. with respect to TMS reference, whereas H + of the OH − ion appears at −0.8 p.p.m. in C12A7. Nearly, the same areal intensities of the spectra further confirm full incorporation of H − and OH − ions. In S12A7, the difference between the values of δ iso for H − (+6.1 p.p.m.) and OH − ions (−1.3 p.p.m.) expands with cage size. Overall, δ iso for H − , δ iso (H − ), is thought to become more positive as the cage size increases and, at the same time, δ iso for H + , δ iso (H + ), becomes more negative. Interestingly, the two values of δ iso (H − ) are outside their typical ranges and apparently reversed compared with the typical positions for protons and metallic hydrides. Indeed, usually δ iso (H + ) varies from +20 to 0 p.p.m. (ref. 32 ), whereas metallic hydrides, such as TiH 2 , typically exhibit δ iso (H − ) below 0 p.p.m. (ref. 28 ). Our data suggest that electron density should be larger around H + than around H − nuclei, provided that the chemical shift is predominantly determined by the chemical shielding effect. This relationship contradicts the formal number of electrons associated with H + (no electrons) and H − (two electrons). Furthermore, our results for hydrogen show opposite behaviour to the NMR spectra of alkali elements. According to the NMR spectra of alkali-organic complexant alkalides, alkali ions such as Na + and K + have positive chemical shifts, whereas alkalide ions such as Na – and K – exhibit relatively negative shifts [34] , [35] . This relationship can be easily understood from the difference in the occupation numbers of the outer s shell, for example, [Ne]3 s 0 for Na + and [Ne]3 s 2 for Na − . Clearly, the same logic does not apply to H + and H − ions. Figure 3: 1 H nuclear magnetic resonance (NMR) spectroscopy. Experimental 1 H-magic-angle-spinning NMR spectra for ( a ) C12A7:H − (red line) and C12A7:OH − (blue line), and ( b ) S12A7:H − (red line) and S12A7:OH − (blue line) samples, and corresponding theoretical spectra for ( c ) C12A7 and ( d ) S12A7 systems. Broad signals between +7 and −2 p.p.m. in the experimental spectra of S12A7 are attributed to adsorbed water and hydroxide impurities. Full size image These experimental results were corroborated with ab initio calculations using the periodic and embedded cluster approaches [16] , [21] , [36] , [37] . Geometrical parameters and NMR chemical shifts were calculated for 12 configurations of H − and OH − ions in C12A7 and S12A7 (for details, see Supplementary Table 7 and Supplementary Note 4 ). The calculated geometrical parameters are very close to those determined experimentally. In particular, the distances between the pole cations agree with those evaluated from XRD data within 1–16 pm, whereas the calculated d O–H…O distance is within 10 pm of the corresponding experimental values. The chemical shifts were calculated using a procedure suggested by Cheeseman et al. [38] that has produced reliable values for the chemical shifts of molecular species. The calculated chemical shifts are in a very good agreement with the experimental data ( Table 1 and Fig. 3 ) and, importantly, they confirm that δ (H − )> δ (H + ). The latter is attributed to the difference of the electron density on the hydrogen nucleus: ρ (H − )< ρ (H + ) in both C12A7 and S12A7. The interaction of a spin-1/2 nucleus (such as 1 H) with its surroundings can be described using the Hamiltonian, H int = H D + H CS + H P + H K + … , which includes the magnetic dipolar interaction, H D ; the chemical shielding effect, H CS ; the paramagnetic spin interaction, H P , and the Knight shift effect, H K (refs 28 , 33 ). The negative δ iso of metallic hydrides is principally ascribed to the Knight shift effect, because of the interaction of nuclear spin with conduction electrons, which introduce an ‘extra’ effective field at the nuclei. Its typical value ranges from 0 to −250 p.p.m. for 1 H (ref. 28 ). Both C12A7:H − and S12A7:H − samples have measurable electrical conductivities because of residual electrons. However, the primary conductivity mechanism is thermally activated polaron hopping [21] , and hence the Knight shift effect can be ruled out. Contribution from H P is also negligible, because the chemical shift is barely affected by the concentration of residual electrons: shifts of less than 0.1 p.p.m. were observed for the electron concentration range of 2 × 10 19 −8 × 10 20 cm −3 (ref. 18 ; Supplementary Fig 1 ). Thus, chemical shielding has the dominant effect on the δ iso (H − ) value. It follows that the electron density around the nucleus is higher for H + than H − ions in mayenites. Effect of structural parameters on chemical shift It is well established that the δ iso (H + ) value has a close relationship with the d O–H…O value [30] , [31] , [39] . The values of δ iso (H + ) observed for the two mayenites also follow this general trend, as shown in Fig. 4 . The fact that δ iso (H + ) in mayenites are negative with respect to TMS is consistent with exceptionally large d O–H…O values. Similarly, we found a correlation between δ iso (H − ) and the distance between the H − ion and its nearest coordinating cation, d M–H . To focus on the electron shielding effect on δ iso (H − ) only, we consider ionic hydrides [40] , [41] , [42] and mixed-anion hydrides [7] , [8] , in which H − ions are coordinated with only saline (alkaline-earth or alkali metals) cations. Their δ iso (H − ) values are plotted against d M–H in Fig. 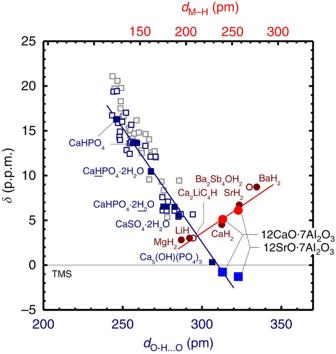4 , and are approximated to a linear function. Figure 4: Dependence ofδisoondO–H…OanddM–H. Data for mayenites are co-plotted with literature data: filled squares for CaO-based compounds31; blue open squares for silicate glasses39; grey open squares for some solid salts30; filled circles for binary saline hydrides with alkaline-earth metals40, Mg41and Li42; open circles for Ca3LiC3H (ref.7) and Ba8Sb4OH2(ref.8). Horizontal axes ofdO–H…OanddM–Hwere adjusted so that each of the two sets of mayenite data were aligned. Taking account of the scattering of data, this relationship can be described as: Figure 4: Dependence of δ iso on d O–H…O and d M–H . Data for mayenites are co-plotted with literature data: filled squares for CaO-based compounds [31] ; blue open squares for silicate glasses [39] ; grey open squares for some solid salts [30] ; filled circles for binary saline hydrides with alkaline-earth metals [40] , Mg [41] and Li [42] ; open circles for Ca 3 LiC 3 H (ref. 7 ) and Ba 8 Sb 4 OH 2 (ref. 8 ). Horizontal axes of d O–H…O and d M–H were adjusted so that each of the two sets of mayenite data were aligned. Full size image To rationalize the observed results, we considered two model systems ( Fig. 5a,b ): (i) a cluster comprising two planar Mg 2 O 2 blocks, sandwiching an OH − ion, was used to investigate the dependence of δ iso (H + ) on d O–H…O and (ii) an H − ion occupying anion site in the bulk of a rock-salt lattice, such as that of MgO, was used to investigate the dependence of δ iso (H − ) on d M–H . The results of these calculations summarized in Fig. 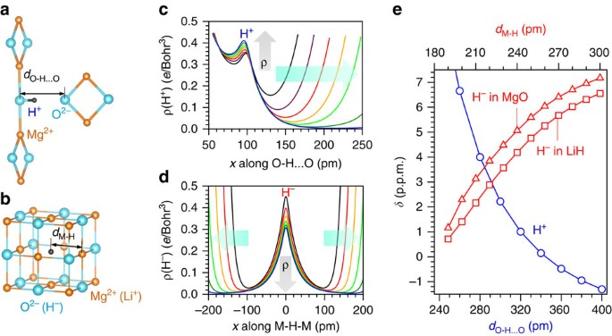5e reproduce well the general trends observed for the H − and OH − ions experimentally. Figure 5: Dependence ofδiso(H+) andδiso(H−) on the characteristic parameters of proton local environment. Model systems are: (a) OH−ion sandwiched between two Mg2O2clusters and forming a hydrogen bond with another Mg2O2cluster, (b) an H−ion at the anion site in the bulk of a rock-salt ionic crystal, such as MgO or LiH. (c) Electron density along the O–H bond of an OH−ion for several values ofdO–H…Oplotted against distance from O atom of the OH−ion. Black to blue lines correspond todO–H…Ovalues of 220, 240, 260, 280, 300, 340 and 400 pm. (d) Electron density along the Mg–H bond of an H−ion in MgO for several values ofdM–H. Black to blue lines correspond todM–Hvalues of 200, 220, 240, 260, 280 and 300 pm. (e) Dependences ofδiso(H+) andδiso(H−) ondO–H…O(circles) anddM–H(triangles for M=Mg and squares for M=Li), respectively. Light-green arrows in (c) and (d) indicate increasing volume associated with hydrogen species, while grey arrows indicate the corresponding change of the charge density magnitude at the hydrogen site. Figure 5: Dependence of δ iso (H + ) and δ iso (H − ) on the characteristic parameters of proton local environment. Model systems are: ( a ) OH − ion sandwiched between two Mg 2 O 2 clusters and forming a hydrogen bond with another Mg 2 O 2 cluster, ( b ) an H − ion at the anion site in the bulk of a rock-salt ionic crystal, such as MgO or LiH. ( c ) Electron density along the O–H bond of an OH − ion for several values of d O–H…O plotted against distance from O atom of the OH − ion. Black to blue lines correspond to d O–H…O values of 220, 240, 260, 280, 300, 340 and 400 pm. ( d ) Electron density along the Mg–H bond of an H − ion in MgO for several values of d M–H . Black to blue lines correspond to d M–H values of 200, 220, 240, 260, 280 and 300 pm. ( e ) Dependences of δ iso (H + ) and δ iso (H − ) on d O–H…O (circles) and d M–H (triangles for M=Mg and squares for M=Li), respectively. Light-green arrows in ( c ) and ( d ) indicate increasing volume associated with hydrogen species, while grey arrows indicate the corresponding change of the charge density magnitude at the hydrogen site. Full size image Here, let us consider how d O–H…O affects the δ iso (H + ) value. Figure 5c shows profiles of calculated electron density with varying d O–H…O . The electron density around the proton nuclei increases with increasing distance. When the distance is short, the proton is attracted to the host oxygen, while the negative charge of the counter oxygen pushes the bonding electrons away from the proton. As a result, the electron density around the proton decreases. As d O–H…O increases, the chemical bond of the OH − ion becomes less polarized and its bond length, d O–H , decreases concurrently. Both factors lead to higher electron density at the hydrogen site, in turn leading to negative shift. The model used to calculate δ iso (H + ) ( Fig. 5a ) reproduces the structure of mayenite cages well, in which two pole cations sandwich an OH − ion. In general, the polarization of an O–H bond is affected not only by the distance d O–H…O but also by ligand ions. When cations are located near the proton, they tend to shorten the O–H bond, which in turn causes an additional negative shift; the effect is opposite for anions. Different ligands from each crystal structure may influence the relationship between d O–H…O and δ iso (H + ). This is discussed in Supplementary Note 5 . As for the H − ion, Fig. 5d demonstrates that as d M–H increases, the electron density around the hydrogen nucleus decreases, inducing the positive chemical shift. The sensitivity of the electron density to d M–H is ascribed to the large polarizability of the H − ion. In general, the site volume for an H − ion increases markedly as the bond character in metal hydrides changes from covalent to ionic [29] . In contrast, saline cations become more electropositive as their radius increases, leading to formation of a bond with more ionic character to the H − ion [29] , [43] . Therefore, the general dependence of δ iso (H − ) on d M–H ( Fig. 4 ) can be explained from the fact that a longer d M–H gives the H − ion more space, which in turn decreases the electron density around the nucleus and moves δ iso (H − ) to a more positive value. The dependence of the δ iso values on the lattice structural parameters discussed above ( Fig. 4 ) can be used to predict the δ iso values for OH − and H − ions. Because OH − and H − ions can occupy equivalent lattice sites, as is the case in mayenites, the ability to make such predictions has practical importance. When both OH − and H − ions are incorporated at equivalent sites in an oxide host, the NMR signal of H − is in the typical range for hydrogen-bonded H + ions. Hence, it may be difficult to distinguish H + and H − ions solely from their δ iso value. Generally, hydrogen is ubiquitous and forms various configurations of H + in oxides, possibly masking the weak NMR signal of diluted H − ions. This suggests that there may be H − ions present in materials that have been overlooked in NMR spectra. In materials with a site volume similar to that of mayenite, the apparent reversal of chemical shift takes place, facilitating identification of the H − signal. Scouting for H − ions among OH − ions To demonstrate that the relationship between d M–H and δ iso is useful for revealing the existence of H − ions and predicting their chemical shifts and to establish a methodology for identifying H − out of various states of H + that ‘hide’ the H − ions, we considered calcium phosphate apatite [31] , [44] , [45] , [46] , [47] , [48] , [49] . As described below, this material hosts similar sets of anions in its special crystallographic sites as mayenite does. Calcium phosphate apatite generally crystallizes in a hexagonal (space group P 6 3 / m ) or pseudo-hexagonal (more exactly monoclinic with a space group P 2 1 / b ) system and is characterized by an isolated tetrahedron of PO 4 3− and two sites with Ca 2+ ions. One of these (the Ca2 site) forms an array of triangles that run along the c -axis. Its inner space is often called a ‘channel’ and is occupied partially or completely by various kinds of anions. The general formula of the unit cell is [Ca 10 (PO 4 ) 6 ] 2+ ·2 Y − , where brackets refer to a positively charged host lattice that incorporates guest anions: 2 Y − =2F − , 2Cl − , 2OH − or O 2− . F − (ref. 44 ) and O 2− (ref. 46 ) ions are located at the centre of Ca 3 triangles, whereas OH − (refs 31 , 46 ) and Cl − (ref. 44 ) ions are positioned on an off-triangle plane along the c -axis (see Fig. 6a ). Although there have been no reports of incorporation of H − ions in the channel of apatite, it is expected from its analogy to mayenite that H − will be formed when apatite is severely reduced in the presence of hydrogen. Because an H − ion has an ionic radius comparable with F − and O 2− ions, the most feasible site in the apatite crystal to accommodate an H − ion is the centre of the calcium triangle (see Fig. 6a ). A chemical shift of +4.9±2 p.p.m. is predicted from the triangle centre to calcium distance of 234 pm according to the relationship given by equation (1). Similarly, the O–H…O distance of 307 pm for the OH − in the channel gives a chemical shift of +1.0±2 p.p.m., which agrees with experimental values [31] , [45] , [47] ( cf . Fig. 4 ). Figure 6: H − ions in apatites. ( a ) Local structure around the channel in apatite, showing the coordinating ions with OH − and H − ions. ( b ) 1 H − magic-angle-spinning nuclear magnetic resonance (NMR) spectra collected in apatite samples annealed in wet N 2 (indicated by blue lines), in dry O 2 (orange) and with TiH 2 (brown and red). Filled areas highlight the signals assigned to H − ions. ( c ) Infrared transmission spectra measured for the same set of samples. ( d ) Correlation between chemical shifts ( δ iso ) in the NMR spectra and wavenumbers in the infrared spectra. Blue and red shaded areas indicate chemical shift ranges predicted using the d M–H and d O–H…O correlations with δ iso (H − ) and δ iso (H + ), respectively, given in Fig. 4 and equation 1. Full size image Then, we prepared several apatite samples annealed in wet air, dry oxygen and with titanium hydride (see the Methods section). NMR and infrared transmission spectra measured for these samples are displayed in Fig. 6b,c , respectively. The signal around 0 p.p.m. is well known to arise from OH − ions in the channel. However, in contrast to mayenite that exhibits only two distinct signals for H − and H + , many peaks appear in the series of apatite samples. Most of them are associated with O–H stretching bands in the infrared spectra, originating from HPO 4 2− groups (indicated iii and iv in Fig. 6c ) [31] , [47] , [48] in the lattice framework of apatite, complex defects of OH − in CaO precipitates (ii and iii) [49] in some apatite samples as well as channel OH − ions (i) [31] , [45] , [47] . This is consistent with a general relationship that correlates the strength of the hydrogen bond with the shift of the O–H stretching frequency to lower wavenumber [1] . At the same time, the chemical shift moves to lower magnetic field because of the decrease in the electron density around the hydrogen nucleus. An unassigned signal remains at 3.6 p.p.m. (shaded in Fig. 6b ), which is in the range of the prediction for the H − ion in the channel. This signal has not been experimentally reported to date but appears only in the severely reduced samples prepared here, and thus is unambiguously assigned to H − ions. Their concentration is estimated to be one-thirtieth of the theoretical maximum, which makes them very difficult to detect and characterize by diffraction techniques. Beyond mayenites and apatite, many oxide-based crystals possess crystallographic sites for OH − or halide ions, whose exchange with H − ions is expected to be possible and would lead to novel material functions. Identification of such novel H − ions both fully occupying a certain crystallographic site and doped at a dilute level will be now possible using NMR spectroscopy. Mayenite sample preparation and characterization The C12A7:OH − sample was prepared by annealing stoichiometric C12A7 powder in a wet N 2 atmosphere at 900 °C. The OH − ion concentration was controlled to a maximum value of 2.3 × 10 21 cm −3 (ref. 25 ). The C12A7:H − sample was obtained by annealing a Czochralski-refined C12A7 crystal sealed together with TiH 2 in a silica tube at 1,100 °C. The reacted layer formed on the crystal was mechanically removed. Electron spin resonance spectra revealed that the samples do not contain any spin-active species except residual (2 × 10 19 cm −3 ) extraframework electrons. The C12A7:e − sample was obtained by chemical reduction of a C12A7 single crystal using metallic Ti as a reducing agent, as described in ref. 19 . The S12A7:OH − sample was prepared by solid-state reaction of Sr(OH) 2 ·8H 2 O and γ-Al 2 O 3 powders at 800 °C in wet N 2 atmosphere as described in ref. 26 . Thermogravimetry-mass spectrometry measurements showed weight loss of 0.9% upon H 2 O desorption suggesting that the concentration of OH − ions is close to the maximum possible. The S12A7:H − sample was prepared by thermally annealing pressed pellets of S12A7:OH − powder mixed with CaH 2 powder, which were encapsulated in a stainless steel tube with Sweagelok plugs, at 500 °C for 16 days. Residual CaH 2 and side product Ca compounds were removed by dissolving the sample in a solution of 0.1 M NH 4 Cl in methanol. The sample powder was washed several times with pure methanol. Residual extraframework electron concentration was evaluated to be ~1 × 10 19 cm –3 by electron spin resonance. The concentration of H − ions in this sample was evaluated to be 2.0±0.1 × 10 21 cm −3 by volumetry [18] , suggesting nearly full incorporation of H − ions (see Supplementary Note 6 ). Apatite sample preparation and characterization Commercial high-density hydroxyapatite ceramic (Cell yard, Pentax/Asahi techno glass/Hoya, purity of >99%, Ca/P ratio of 1.667) was used as a starting material. The pellets were annealed in dry O 2 atmosphere at 1,200 °C for 4 days (dry oxygen sample) or in wet N 2 at 900 °C for 6 days using a tube furnace (wet N 2 sample). In other batches, the apatite pellets were put in an Ti-foil envelope containing TiH 2 powder, and then the envelope was sealed in an evacuated silica glass capsule. Heat treatment was carried out at 1,000 °C for 4 days (TiH 2 (#1) sample) or 20 days (TiH 2 (#2) sample). After that, the reaction layer formed on the surface was removed by mechanical grinding. infrared transmission spectra were measured with a Perkin-Elmer Spectrum One spectrometer (Perkin-Elmer) using mirror-finished samples with thicknesses of 40–200 μm. Diffractometry Powder XRD patterns for C12A7 samples were collected at 300 K with a diffraction angle range of 4–70° and an incident X-ray wavelength of 0.5016 Å using a Debye-Scherrer camera at beam line BL02B2, SPring-8. The Enigma programme was used for Rietveld/MEM analysis. The powder XRD patterns for S12A7 samples were collected at 298 K with a diffraction angle range of 10–140° using a Rigaku Rint-2000 XRD (Rigaku; Bragg-Brentano geometry, Cu K α source). The Rietan-2000/Prima programme was used for Rietveld/MEM analysis. NPD data were collected for the S12A7:H − sample at 290 K with a diffraction angle range of 10–165° at a wavelength of 1.495 Å using a high-resolution powder diffractometer for thermal neutrons (HRPT, Paul Scherrer Institut). Rietveld analysis was performed using the Rietan-FP programme. The Vesta programme was used to plot all structural models and electron density maps. NMR spectroscopy 1 H NMR spectroscopic measurements were performed on a Bruker Biospin DSX-400 spectrometer (Bruker) operating at a resonance frequency of 400.13 MHz equipped with a high-speed MAS probe with a diameter of 5 mm. Each granulated sample was weighed (about 70 mg) to obtain a quantitative result and sealed in a zirconia rotor. The rotation frequency was 30 kHz. Spectra were acquired with 90° pulses with a duration of 2.5 μs and an interval of 10–100 s. Chloroform (+7.25 p.p.m. with respect to TMS) was used as a secondary reference for the chemical shifts. Theoretical calculations A quantum-mechanically treated cluster, which included a framework cage hosting extraframework H − and OH − ions, was embedded into the rest of C12A7 and S12A7 lattices considered classically. The total energy of these systems was minimized with respect to coordinates of ~500 atoms including the quantum-mechanically treated cluster and its surrounding. Density functional theory and the hybrid B3LYP density functional, as implemented in the Gaussian 03 package [37] , together with the 6-31 G(d) basis set, were used for the geometry optimization. Then, chemical shifts were calculated using two hybrid density functionals, the Hartree–Fock method and the 6-311+G(2d,p) basis set [38] (see Supplementary Notes 5 and 6. ). How to cite this article: Hayashi, K. et al. Hydride ions in oxide hosts hidden by hydroxide ions. Nat. Commun. 5:3515 doi: 10.1038/ncomms4515 (2014).